Genetic similarity between cancers and comorbid Mendelian diseases identifies candidate driver genes Despite large-scale cancer genomics studies, key somatic mutations driving cancer, and their functional roles, remain elusive. Here, we propose that analysis of comorbidities of Mendelian diseases with cancers provides a novel, systematic way to discover new cancer genes. If germline genetic variation in Mendelian loci predisposes bearers to common cancers, the same loci may harbour cancer-associated somatic variation. Compilations of clinical records spanning over 100 million patients provide an unprecedented opportunity to assess clinical associations between Mendelian diseases and cancers. We systematically compare these comorbidities against recurrent somatic mutations from more than 5,000 patients across many cancers. Using multiple measures of genetic similarity, we show that a Mendelian disease and comorbid cancer indeed have genetic alterations of significant functional similarity. This result provides a basis to identify candidate drivers in cancers including melanoma and glioblastoma. Some Mendelian diseases demonstrate ‘pan-cancer’ comorbidity and shared genetics across cancers. Recent years have brought an explosion in the number of genomically profiled tumours, and the promise of finding most genetic loci containing cancer-predisposing variation seems within reach. Although algorithms to sort through the complex landscape of tumour lesions [1] , [2] have revealed recurrently altered ‘driver loci’—those somatic or germline genetic defects that are most likely to trigger the disease—the directory of relevant genes and the catalogue of their roles in tumour progression remain incomplete. The search for cancer genes has expanded to additional informative patterns, such as mutual exclusivity of mutation across patients and functional relationships between cancer-altered genes [3] , [4] , [5] . One historical source of information on key cancer alterations may be found in Mendelian disorders, rare conditions that have long provided insight into a wide array of human disease processes. Some of the first genes linked to cancer were characterized by their highly penetrant familial association with certain tumours. Studies of familial retinoblastoma led to the identification of RB1 as a tumour suppressor [6] , whereas cases of Li-Fraumeni syndrome showed that germline mutation of TP53 pleiotropically predisposes patients to many cancers [7] . Other Mendelian disorders, such as Rubinstein–Taybi syndrome, involve a primary phenotype apparently unrelated to cancer, yet the bearers are known to have an increased tumour risk [8] . Recent studies demonstrating that Rubinstein–Taybi’s primary causative gene, CREBBP , is also recurrently somatically inactivated in a number of cancers [9] , [10] , [11] have provided a likely explanation for this comorbidity. These examples suggest that Mendelian germline mutations could predispose Mendelian disease patients to common cancer by disrupting cellular functions that in the majority of cancer patients are altered by somatic rather than germline genetic events. Recently, Electronic Health Record (EHR) data sets of unprecedented size have provided statistical power to measure comorbidity of pairs of diseases [12] , [13] , [14] . With the recent increase in the amount of data recorded in EHRs, it is newly possible to detect clinical associations even in diverse rare diseases, such as some Mendelian diseases. These results have suggested that comorbidity is indicative of shared germline genetic architecture. Here, we propose that Mendelian disease comorbidity with cancer could be associated with a relationship between Mendelian disease loci and driver loci somatically altered in cancer. It is possible that genetic variants that cause Mendelian disease with high cancer comorbidity also provide a selective advantage to aberrant cells of a developing tumour, leading to this predisposition to a certain type of cancer. If this is correct, exactly the same Mendelian loci and molecular pathways incorporating their products would be involved in a somatic context in tumours of patients lacking the germline mutation. Thus, comorbidity calculated from EHRs spanning large numbers of patients could provide a novel line of evidence for functional involvement of some genes as cancer drivers. By integrating clinical data from more than 100 million patients with somatic genomic information from thousands of tumours from The Cancer Genome Atlas (TCGA) [15] , we explore genetic relationships between Mendelian diseases and common cancers. First, we examine the hypothesis that comorbidity between Mendelian disease and cancer may be due to similarities between the genes involved in each. We find that comorbid diseases have statistically significant genetic similarity. Having established this association, we test for genetic similarity of comorbid pairs of Mendelian disease and cancer, identifying disease pairs with shared cellular processes. For each TCGA cancer type, we identify genes from comorbid and genetically similar Mendelian diseases as candidate cancer drivers. Integration of disease comorbidities and genes In the work of Blair et al. [14] , the authors estimated comorbidity among a set of diseases well characterized by patient billing codes, comprising 95 Mendelian diseases and 65 complex diseases, including 13 common cancers. Comorbidity was calculated using seven EHR data sets, including the MarketScan insurance claims database covering nearly 100 million patients. For each complex disease, they compared its incidence in Mendelian disease patients against its marginal incidence. Patient zip code information was connected with US census data to obtain demographic, socioeconomic and environmental factors. They then corrected for these confounders, as well as for errors in billing codes, using a regression approach. Combining these analyses, they estimated relative risk for a complex disease in Mendelian disease patients. We use these estimates throughout this work. For each Mendelian disease billing code set, the authors curated a list of corresponding diseases, each linked to genetic loci [16] . Utilizing their work and other curation, we find a median of four genes related to each Mendelian disease type (the full distribution is shown in Supplementary Fig. 1a , and the genes associated with each disease is available in Supplementary Data 1 ). Of the 13 cancer diagnosis code sets included in the Blair analysis, 10 correspond to one or more tumour types profiled in TCGA ( Supplementary Data 2 ). These 10 diagnosis codes correspond to 15 TCGA tumour types, including melanoma, glioblastoma and other common cancers, with genomic data across a total of 5,667 patients. For each tumour type, we gather sets of genes identified as significantly mutated by MutSig [1] or located in peaks of copy-number amplification or deletion by GISTIC2 (ref. 2 ; Fig. 1a ). A median 155 genes are recurrently genetically altered per tumour type ( Supplementary Fig. 1b ). 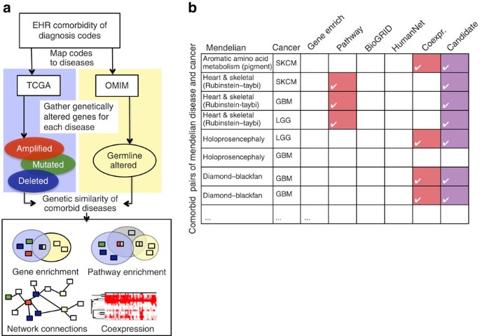Figure 1: Outline of the approach. (a) Integration of the data and overview of genetic similarity metrics. (b) Examples of comparison of pairs of diseases. All comorbid pairs of Mendelian disease and cancer with TCGA data are compared. Genetic similarity of comorbid diseases is assessed using multiple metrics. A simple combination of presence of any one of the genetic similarity metrics is used to predict novel cancer driver loci in the comorbid disease pairs. coexpr., coexpression. Figure 1: Outline of the approach. ( a ) Integration of the data and overview of genetic similarity metrics. ( b ) Examples of comparison of pairs of diseases. All comorbid pairs of Mendelian disease and cancer with TCGA data are compared. Genetic similarity of comorbid diseases is assessed using multiple metrics. A simple combination of presence of any one of the genetic similarity metrics is used to predict novel cancer driver loci in the comorbid disease pairs. coexpr., coexpression. Full size image Investigating genetic similarity between comorbid diseases To assess whether comorbid Mendelian diseases and common cancers share similar genes and cellular processes, we compare the sets of genes associated with a Mendelian disease to the recurrently genetically altered genes in TCGA. We consider multiple measures of genetic similarity, reflecting different potential relationships, including (1) shared genes, (2) shared pathways and (3) gene and protein interactions. We show that comorbid disease pairs have significantly more genetic similarity than expected at random. First, we examine whether the genes responsible for a Mendelian disorder are more likely to be altered in comorbid cancers. For each of the 427 pairs of comorbid Mendelian disease and TCGA cancer, we assess how many genes are shared. Across all comorbid pairs, 41 genes are shared between the Mendelian causal gene set and the recurrently somatically altered cancer gene set ( Fig. 2a ), while 29 would be expected ( P =0.021, as described in Methods and shown in Supplementary Fig. 2a ). 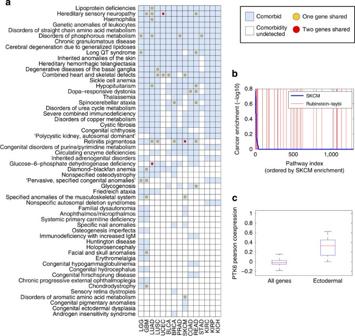Figure 2: Illustration of genetic similarity comparisons in comorbid diseases. (a) The number of genes shared in comorbid diseases is counted across all pairs. By comparing it to a null distribution on the basis of number of Mendelian and cancer genes, we can assess if more genes are shared than expected. Cancer abbreviations are inSupplementary Data 2. (b) For a disease pair, the pathway metric compares the pathways impacted by the Mendelian disease to the pathways enriched for the cancer gene sets. Here, pathway enrichments for melanoma genes (blue) are compared with pathways involved in Rubinstein–Taybi syndrome. Each vertical red line represents one pathway impacted by a Rubinstein–Taybi gene. The pathways are sorted by their enrichment in melanoma. The Spearman correlation between the correctedPvalues of melanoma and the impacted pathways of Rubinstein–Taybi for the pathways is −0.25,P=6.3 × 10−21. (c) Coexpression of all genes (n=17,705) withPTK6,a recurrently amplified gene in melanoma, versus the coexpression of the genes associated with the comorbid disease set ectodermal dysplasias including epidermolysis bullosa (n=15). Outliers are removed, box and whiskers show median and 25th to 75th percentiles. The two-tailed rank-sumPvalue, controlled for number of cancer genes, is 2.0 × 10−6. Figure 2: Illustration of genetic similarity comparisons in comorbid diseases. ( a ) The number of genes shared in comorbid diseases is counted across all pairs. By comparing it to a null distribution on the basis of number of Mendelian and cancer genes, we can assess if more genes are shared than expected. Cancer abbreviations are in Supplementary Data 2 . ( b ) For a disease pair, the pathway metric compares the pathways impacted by the Mendelian disease to the pathways enriched for the cancer gene sets. Here, pathway enrichments for melanoma genes (blue) are compared with pathways involved in Rubinstein–Taybi syndrome. Each vertical red line represents one pathway impacted by a Rubinstein–Taybi gene. The pathways are sorted by their enrichment in melanoma. The Spearman correlation between the corrected P values of melanoma and the impacted pathways of Rubinstein–Taybi for the pathways is −0.25, P =6.3 × 10 −21 . ( c ) Coexpression of all genes ( n =17,705) with PTK6, a recurrently amplified gene in melanoma, versus the coexpression of the genes associated with the comorbid disease set ectodermal dysplasias including epidermolysis bullosa ( n =15). Outliers are removed, box and whiskers show median and 25th to 75th percentiles. The two-tailed rank-sum P value, controlled for number of cancer genes, is 2.0 × 10 −6 . Full size image Second, we test the hypothesis that comorbid diseases share common cellular processes. For this purpose, we count the shared pathways between comorbid diseases, using 1,343 pathway gene sets compiled in the Consensus Pathway Database [17] . A pathway is considered shared if it is enriched for the cancer gene set and contains a Mendelian disease gene. Aggregating across all comorbid pairs, we find 136 shared pathways, while 65 would be expected ( P <10 −5 , using convolution of hypergeometric distributions as described in Methods, and shown in Supplementary Fig. 2b ). Third, we test the hypothesis that the number of direct interactions between Mendelian disease genes and genes somatically mutated in comorbid cancer is elevated, using established gene interaction networks. We compare the observed number of interactions in a network against a null model comprised of a set of randomly shuffled networks, controlling for the number of network edges each gene has. We test this measure in two interaction networks. The first network, BioGRID [18] , is a large curated network of protein and genetic interactions. We observe 797 direct edges in this network, more than 98.3% of random networks ( Supplementary Fig. 2c ). The second network, HumanNet [19] , contains uncurated connections generated from integrated data sources. We find 296 connections, which is more than in 99.8% of the random networks ( Supplementary Fig. 2d ). Note that to assess the significance of novel Mendelian disease associations with cancer, this analysis excludes well-known Mendelian cancer syndromes (Li–Fraumeni syndrome, specified hamartoses, multiple endocrine neoplasia, neurofibromatosis and tuberous sclerosis). These cancer syndromes, as would be expected, are each comorbid with multiple cancers, and they show many shared genes and pathways with the cancers ( Supplementary Data 3 ). Thus, using a number of lines of evidence, we have shown that the genes involved in Mendelian diseases have statistically significant genetic similarity with the genes altered in co-occurring cancers. Therefore, comorbidity may be due to these shared genetic processes. Interestingly, most of these connections have not been not previously reported. Prediction of diseases with shared cellular processes To use comorbidity as a way of identifying candidate drivers for each cancer, we apply a version of the previously described metrics to each pair of comorbid diseases. Just as we tested for a significant number of genes shared across all comorbid disease, we perform a similar test for each pair of Mendelian disease and cancer. This gene-enrichment metric assesses overrepresentation of the set of Mendelian disease genes within the somatically altered cancer gene set. For the pairwise shared pathway metric, we assess whether the pathway-enrichment scores are significantly correlated for the pair of diseases ( Fig. 2b ). The network metric tests whether a Mendelian disease gene set has more direct interactions with a set of comorbid cancer genes than the random expectation, testing interactions from BioGRID and HumanNet separately. In addition, to test for functional similarity in an unbiased fashion, we compare coexpression of Mendelian and cancer genes. We use a large and diverse panel of human primary cells, tissues, and cell lines from the FANTOM5 project [20] . For each pair of diseases, we test whether any cancer-altered genes show significantly elevated coexpression with the set of Mendelian disease genes ( Fig. 2c ). After correcting for the number of comorbid pairs (see Methods), we find that coexpression has the most instances of similarity, most likely due to the fact that more genes can be compared and many types of functional relationships can be captured with coexpression. In contrast, the gene enrichment and network metrics have very few instances of significant similarity, a point that is discussed below. These metrics define a list of candidate driver genes. The complete list of genes and genetic similarity scores associated with each linked disease pair is available in Supplementary Data 4 . To provide examples and to demonstrate their relevance, we highlight some candidates implicated for cutaneous melanoma and brain neoplasms. Cutaneous melanoma is often located on sun-exposed sites, undergoing a high rate of genetic damage. Our findings highlight both recurrently altered genes in melanoma and comorbid Mendelian genes as potential cancer drivers. A central transcription factor involved in melanocyte cell fate, MITF, is related to multiple Mendelian diseases comorbid with melanoma. This gene has a complex role in this cancer: while it is recurrently amplified in 26% of TCGA melanomas, possibly promoting melanocyte proliferation, it is also frequently deleted (11% of cases). Suppression of the gene is also advantageous for the growing cancer, as it reduces terminal differentiation and senescence in melanocytes [21] , [22] . The melanocyte’s primary receptor MC1R, upstream of MITF, its other upstream activators, PAX3 and SOX10, as well as MITF’ s key target, TYR, are all associated with Mendelian disorders comorbid with melanoma ( Fig. 3a ). 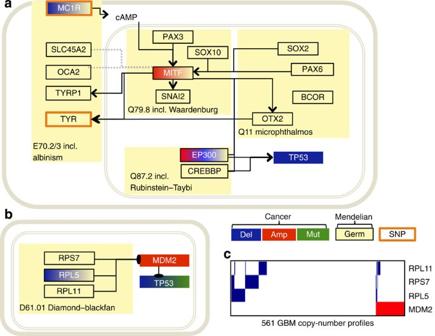Figure 3: Examples of comorbid Mendelian diseases in melanoma and glioblastoma. (a) Depiction of comorbid diseases with skin melanoma, in terms of the roles of the Mendelian disease genes in the melanocyte development program as well as other cancer-related processes. Genes that are recurrently somatically mutated in melanoma are highlighted. Solid edges represent interactions from the literature, while the dashed edges represent significant coexpression. (b) Interaction of Diamond–Blackfan anemia genes with glioblastoma altered genes. (c) Summary of copy-number changes toMDM2and the Diamond–Blackfan associated ribosomal proteins known to suppress the action ofMDM2. Among the ribosomal genes,RPL5is recurrently and focally deleted such as to be in the GISTIC2 results, and it shows mutual exclusivity withMDM2amplification (one-tailed Fisher’s exact test,P=0.033).RPL11deletion also has mutual exclusivity withMDM2amplification (P=0.042).RPS7andRPL11deletions, together withRPL5deletions, form a weaker mutually exclusive trend withMDM2(P=0.060). amp, amplification; del, deletion; germ, germline; incl., including; mut, mutation; SNP, single-nucleotide polymorphism. Figure 3: Examples of comorbid Mendelian diseases in melanoma and glioblastoma. ( a ) Depiction of comorbid diseases with skin melanoma, in terms of the roles of the Mendelian disease genes in the melanocyte development program as well as other cancer-related processes. Genes that are recurrently somatically mutated in melanoma are highlighted. Solid edges represent interactions from the literature, while the dashed edges represent significant coexpression. ( b ) Interaction of Diamond–Blackfan anemia genes with glioblastoma altered genes. ( c ) Summary of copy-number changes to MDM2 and the Diamond–Blackfan associated ribosomal proteins known to suppress the action of MDM2 . Among the ribosomal genes, RPL5 is recurrently and focally deleted such as to be in the GISTIC2 results, and it shows mutual exclusivity with MDM2 amplification (one-tailed Fisher’s exact test, P =0.033). RPL11 deletion also has mutual exclusivity with MDM2 amplification ( P =0.042). RPS7 and RPL11 deletions, together with RPL5 deletions, form a weaker mutually exclusive trend with MDM2 ( P =0.060). amp, amplification; del, deletion; germ, germline; incl., including; mut, mutation; SNP, single-nucleotide polymorphism. Full size image Of these, MC1R and TYR are associated with oculocutaneous albinism (included in International Classification of Disease, revision 10 (ICD10) billing code E70.2/3, melanoma relative risk 95% confidence interval (CI)=(2.16–5.19)). MC1R is among the recurrently deleted genes in melanoma. Germline variants of MC1R, causing red hair, have been implicated as a risk factor for melanoma via both pigmentary and non-pigmentary pathways [23] , [24] , and polymorphic variants of TYR, which leads to green eyes, also confer significant, though lesser, risk [25] . Other albinism-related genes have significantly elevated coexpression with MITF (corrected rank-sum P =0.020) as well as MITF' s target gene [26] KCNAB2 (corrected rank-sum P =0.0093) . KCNAB2 is recurrently deleted in the melanoma cases. Although the candidate melanoma genes associated with albinism are not recurrently genetically mutated in melanoma, we examine their patterns of expression for evidence of a functional contribution to the disease. Clustering melanoma tumours by their expression of these genes, we find stable clusters ( Supplementary Fig. 3a ). We assess clinical outcome in these groupings, and we find that the cluster assignments are highly predictive of patient survival ( P =0.0022, Supplementary Fig. 3b ). This suggests that indeed this pathway is highly relevant for melanoma progression. Also regulating MITF activity are its coactivators EP300 and CREBBP [27] , genes associated with the melanoma-comorbid Rubinstein–Taybi syndrome (code group Q87.2, relative risk 95% CI=1.19–1.99). EP300 is recurrently amplified (36% of the TCGA melanomas), but also frequently deleted (7% of cases). Rubinstein–Taybi shares many pathway with melanoma ( Fig. 2b ), including ‘melanocyte development and pigmentation’ and ‘regulation of nuclear beta catenin signaling and target gene transcription’, both of which involve MITF . The amplifications of EP300 are significantly more likely to co-occur in the same patients with MITF amplifications (one-tailed Fisher’s exact test, P =0.0041), suggesting cooperation between the alterations, and a particular role for these genes in melanoma: the histone acetyltransferase activity of EP300 might enhance the function of an oncogenically amplified MITF . CREBBP and EP300 defects have also been linked to aberrant TP53 and BCL6 regulation in some lymphomas [28] . Comorbidity of melanoma with ectodermal dysplasias (ICD10 code Q81, melanoma relative risk 95% CI=6.01–17.84) may highlight the importance of tissue invasion in melanoma progression. The ectodermal dysplasia disease epidermolysis bullosa can arise from genetic alteration to proteins involved in structural support, tissue integrity and adhesion in the dermis and epidermis. Although the chronic inflammation and tissue damage associated with epidermolysis bullosa may play a role in its known risk for skin cancers, subtypes of the condition have been shown to lead to skin squamous cell carcinoma that is more aggressive than in other conditions involving chronic skin scarring [29] . The ectodermal dysplasia genes show high coexpression with melanoma-altered genes related to cell contact in the epithelium, especially PTK6 ( Fig. 2c ). This gene is focally amplified in 44% of melanomas and has an identified role in epithelial invasion and mesenchymal transition in prostate and breast cancers [30] , [31] , but PTK6 has been rarely studied in melanoma. The TCGA melanoma cohort is primarily composed of metastasis samples, but the expression data also includes 103 primary tumours, mostly stage IIC, along with 368 metastases. As changes in cell contact and mesenchymal transition may be related to metastasis state, we compare expression in primary versus metastasis. We find that PTK6 is significantly differentially expressed (adjusted P -value=3.29 × 10 −28 ). In addition, of 11 ectodermal dysplasia candidate melanoma genes, nine are significantly downregulated in metastases as compared with primary (gene set differential expression camera P value=0.00032, GSEA P value=0, Supplementary Fig. 4 ). The other cancers included in our study also have informative genetic and clinical links with Mendelian disease. Diamond–Blackfan anemia, a blood disorder, is comorbid with the brain neoplasms (ICD10 D61.01, relative risk 95% CI=9.22–28.67). Indeed, Diamond–Blackfan patients have risk for seven of the cancer ICD-9 code groups, along with other blood and solid cancers [32] . Among Diamond–Blackfan’s causal genes is RPL5, a gene that is significantly deleted in 8% of TCGA glioblastoma and that suppresses MDM2 (ref. 33 ; Fig. 3b ). MDM2 is recurrently amplified in 15% of TCGA glioblastoma cases. It is an established oncogene that negatively regulates TP53 (ref. 34 ). Like RPL5, other Diamond–Blackfan genes RPL11 and RPS7 repress MDM2 in response to ribosomal stress [34] . The deletion of RPL5 is mutually exclusive with amplification of MDM2 ( P =0.033, Fig. 3c ), supporting the role of RPL5 deletion as an alternative mode of TP53 abrogation. While RPL11 is less frequently deleted, it also has a mutually exclusive pattern with MDM2 amplification ( P =0.042). The role of these ribosomal proteins in glioblastoma appears to be unstudied, making this a strong candidate for further study. Although Diamond–Blackfan anemia is comorbid with many cancers, the cranial development disorder holoprosencephaly is comorbid only with the brain neoplasms (ICD10 Q04.2, relative risk 95% CI=9.30–15.95). Defects in genes that regulate cranial-specific components of the sonic hedgehog pathway are responsible for the improper embryonic patterning in holoprosencephalies [35] . This pathway regulates expression of the GLI transcription factors, which have been linked to maintenance of stemness in gliomas [36] . Subtypes of glioblastoma have been defined on the basis of gene expression patterns, and among these the Classical subtype has a signature including Sonic hedgehog signalling [37] . Holoprosencephaly genes have weak pathway-enrichment similarity with low-grade glioma genes, as well as coexpression with multiple of the low-grade glioma genes, particularly the recurrently copy-number-altered gene VENTX (corrected rank-sum P =0.0092). In the TCGA lower-grade glioma cohort, VENTX lesion occurs more in higher-grade tumours, and these lesions are anticorrelated with IDH1 mutation. Mutation of IDH1 is associated with good prognosis and particularly co-occurs in subtypes of low-grade glioma with either TP53 alteration or 1p19q codeletion [38] . Comparing the IDH1 mutated against the VENTX mutated samples, we find strong differential expression of the holoprosencephaly genes TGIF1, SIX3, ZIC2, GLI2 . As a set, the holoprosencephaly candidate brain neoplasm genes are significantly upregulated in the VENTX mutated tumours (camera P value=0.048, GSEA P value=0.031, Supplementary Fig. 5 ). Both VENTX mutation and activated hedgehog signalling are thus associated with higher-grade gliomas. Changes in regulation of the sonic hedgehog pathway may be an important step in the progression of lower-grade glioma, as in classical glioblastoma. Pan-cancer Mendelian associations Above, we describe a number of processes aberrantly regulated in Mendelian disease and in common cancer. The Blair analysis [14] suggested that the unique set of Mendelian diseases comorbid with a complex disease represented a sort of barcode, indicative of the unique set of cellular processes underlying each disease. This hypothesis is indeed reflected in the sets of disorders, and underlying genetic lesions, found in this study. On the other hand, some Mendelian diseases predispose carriers to many cancer types, while others have no relationship with cancer. In fact, the number of comorbid cancers per Mendelian disease follows a highly non-random distribution ( Fig. 4a ). One interpretation of this pattern is that the genes altered in some Mendelian diseases, such as Li–Fraumeni syndrome, Rubinstein–Taybi syndrome and Diamond–Blackfan anemia, are related to pan-cancer processes common to cancer development in many contexts. This interpretation is supported foremost by our finding of statistically significant genetic similarity in comorbid disease pairs. In addition, we examine four new cancers with available TCGA data but no comorbidity information (ovarian, thyroid, head and neck, and acute myeloid leukemia). If the pan-cancer Mendelian diseases impact core cancer processes, we would expect these to be relevant to these new cancers. We test whether pathways associated with Mendelian diseases with many (more than five) cancer comorbidities are enriched in the four new cancers. We find that the Mendelian diseases with multiple comorbidities share 27 pathways with the four cancers with no comorbidity information, more than the random expectation ( P =0.005, excluding Mendelian cancer syndromes). In another test of this hypothesis, we assess whether Mendelian diseases with more cancer comorbidities are associated with genes that have cancer-related characteristics. We create a set of the 48 genes recurrently altered in more than four of the 19 TCGA tumour types. We call these the multi-cancer mutation genes. Examining FANTOM5 coexpression of the Mendelian disease genes and the multi-cancer mutation genes, we find a significant correlation with number of cancer comorbidities in the gene's associated Mendelian disease. That is, the more the cancers are comorbid with a Mendelian disease, the higher the coexpression of a Mendelian disease gene and multi-cancer mutation genes (Spearman correlation P value=0.027). These findings suggest that some Mendelian diseases predispose patients to many cancers by genetic alterations affecting pan-cancer processes. 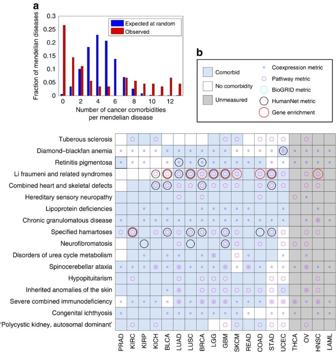Figure 4: Some Mendelian diseases appear to have pan-cancer comorbidity and genetic similarity. (a) The distribution of the number of comorbid cancer diagnosis codes per Mendelian disease is shown. The actual distribution (red bars) includes a large number of Mendelian diseases with no cancer relationship, and a long tail with Mendelian diseases that are comorbid with many cancers. The blue bars represent the expected distribution: about one-third of the pairs of disease have a comorbidity relationship, thus the expected mode of the distribution would have four comorbid cancers per Mendelian disease. The expected distribution is modelled using a binomial. (b) Mendelian diseases that have comorbidity with and genetic similarity to more than three cancers are compared with all 19 available TCGA cancers, 15 of which have comorbidity information. These mostly have widespread comorbidity and show genetic similarity (after multiple testing correction) across many cancers. Similarity was calculated here without removing the known germline-associated cancer genes to view all the associations. Figure 4: Some Mendelian diseases appear to have pan-cancer comorbidity and genetic similarity. ( a ) The distribution of the number of comorbid cancer diagnosis codes per Mendelian disease is shown. The actual distribution (red bars) includes a large number of Mendelian diseases with no cancer relationship, and a long tail with Mendelian diseases that are comorbid with many cancers. The blue bars represent the expected distribution: about one-third of the pairs of disease have a comorbidity relationship, thus the expected mode of the distribution would have four comorbid cancers per Mendelian disease. The expected distribution is modelled using a binomial. ( b ) Mendelian diseases that have comorbidity with and genetic similarity to more than three cancers are compared with all 19 available TCGA cancers, 15 of which have comorbidity information. These mostly have widespread comorbidity and show genetic similarity (after multiple testing correction) across many cancers. Similarity was calculated here without removing the known germline-associated cancer genes to view all the associations. Full size image The Mendelian diseases with the most links to cancer indeed impact pathways shared across many cancers, including telomere maintenance, DNA damage response and mTOR signaling ( Fig. 4b , and Supplementary Data 3 and 4 ). Pan-cancer associations with immunodeficiency syndromes could be owing to the compromised immune system, rather than the ability of the tumour to evade immune suppression. However, we find many instances of genetic similarity with cancer, suggesting that the same functions are frequently somatically altered in tumours. For example, the gene B2M is recurrently mutated or deleted in the TCGA melanoma, lung squamous cell carcinoma and colon adenocarcinoma. Loss of this gene leads to abolition of the MHC class I complex in tumour cells and has been shown to influence immune escape in some lymphomas [39] . B2M has significant coexpression with the immunodeficiency genes, and CIITA and RFX5 , immunodeficiency genes that mainly regulate MHC class II expression, have a secondary role in regulating MHC class I expression [40] . Novel pan-cancer associations include the set of lipoprotein deficiencies, defects in widely expressed proteins that lead to an imbalance of blood cholesterols. The genes associated with lipoprotein deficiencies also influence inflammation and are enriched in the highly cancer-relevant TGF-β pathway. Cancers, with their elevated rates of proliferation, are thought to have high cholesterol metabolism, and the role of blood cholesterol in tumour progression is a current area of research [41] . The lipoprotein deficiency genes are significantly coexpressed with a number of metabolism-related genes that are recurrently mutated in multiple cancers ( Supplementary Data 4 ). These include IDH1, a gene that has been shown to be regulated with cholesterol levels [42] and to be relevant in gliomas and other cancers [43] . If pan-cancer Mendelian associations exist, this further supports the hypothesis that comorbidity between Mendelian disease and cancer is owing to shared processes disrupted by germline or somatic alterations, respectively. We have shown that Mendelian diseases that are comorbid with a cancer are likely to involve mutation of genes similar to those that are somatically altered in that cancer. Importantly, this suggests that comorbidity between Mendelian disease and cancer may be due to germline mutations that provide a fertile ground for the growth of certain aberrant cells. This novel finding provides new insight into the somatic genetic alterations present in a cancer, presenting them in the context of well-characterized diseases with simpler genetics. While algorithms for classifying genes as preferentially somatically mutated in a cancer are an active area of research, comorbidity can provide an orthogonal line of evidence for involvement of cellular processes in oncogenesis and pinpoint driver genes among the recurrently mutated genes. Candidate drivers among the Mendelian disease genes include many genes that are less recurrently somatically mutated, but impact the same pathways. Many of our candidate drivers have a bulk of evidence supporting their role: beyond our findings related to comorbidity and genetic similarity, the candidate genes include some recurrently mutated in cancer, and some with identified roles as drivers in other tumours. In addition, we have used patterns of co-occurrence of candidate mutations across tumour cohorts to demonstrate a likely role for these genes in the tumours. For less frequently mutated candidate drivers, we have related gene expression with clinical indicators. Our results are informative of the many processes that are involved in cancer development. Inactivation of ribosomal protein RPL5, associated with Diamond–Blackfan anemia, has the potential to cause aberrant TP53 degradation in multiple cancers. As cancer is known to involve defects in differentiation [44] , much like a number of Mendelian diseases, a role for the Mendelian disease genes in cancer dedifferentiation and aberrant proliferation is plausible. Other ‘hallmarks of cancer’, such as invasion or regulation of apoptosis are also represented in the Mendelian diseases. As cancers have many altered processes in common, it is logical that we also find some ‘pan-cancer’ Mendelian diseases with multiple genetic and clinical associations. In contrast, some germline variants predispose patients to a more narrow range of cancers, which can reveal more specific oncogenic processes. A few Mendelian disorders are comorbid only with brain neoplasms and melanoma. As melanocytes are descended from the neural crest, Mendelian genetic lesions affecting neural development are likely to affect processes in melanocytes, including proliferation and terminal post-mitotic differentiation. One interesting example is microphthalmos, meaning small eye, a disease phenotype that, in the mouse, gave rise to the name of the melanoma oncogene MITF (microphthalmos transcription factor). In humans, the most common causal genes are closely tied in expression and in function to MITF [45] ( Fig. 3a ). Some of the microphthalmos genes have been implicated in neural-derived tumours [46] , [47] , [48] , and these may be exciting novel candidates in melanoma. There is a link between some sensineural disorders and pigment anomalies: the phenotype of microphthalmos can also occur to varying degrees in patients with Rubinstein–Taybi syndrome and in patients with Waardenburg syndrome, a pigment and deafness disorder. The idea that disorders comorbid with the same cancer may share pathways with each other is highly intriguing. Waardenburg syndrome (included in ICD10 code group Q79.8), like microphthalmos, shows comorbidity only with melanoma and brain neoplasms. Waardenburg has correlated pathway enrichment to melanoma ( P =5.8 × 10 −4 ): both diseases are impact melanocyte development and β-catenin signaling pathways. However, the billing code used is not specific enough to have significant enrichment. In fact, many of the Mendelian diseases with an apparent risk for cancer do not display genetic similarity by our pairwise metrics. We chose a limited number of genetic similarity metrics to consider different lines of interpretable evidence for functional similarity, but other comparisons of genetic similarity could capture more connections. For example, the blood disorder thalassemia can lead to overloaded blood iron levels [49] which may explain these patients’ risk for a variety of cancers [50] ; however, this effect is not detected by our current approach. In addition, a number of factors introduce noise into our source data. These issues include ambiguity of the diagnosis codes; heterogeneity of the Mendelian diseases; insufficient sampling of the mutation spectrum of both Mendelian disease and of cancer. Our finding of statistically significant association of genetic similarity with comorbidity, despite these factors, is a main discovery of our work. This implies that future large-scale studies mining rich data sources such as the eMERGE network [51] will find more genetic and clinical associations. Other future work building on our results includes, foremost, the experimental assessment of the candidate driver genes. Drugs that target these cellular processes, perhaps as studied in Mendelian disease patients, may be applicable for the treatment of the tumours [52] . Data sets We used the Supplementary Material available in Blair et al. [14] , to classify pairs of Mendelian disease and complex disease as having a comorbidity relationship. In that study, the authors curated Mendelian diseases, and their corresponding genes from the Online Mendelian Inheritance in Man (OMIM) [16] , and mapped them to ICD code sets, which they assessed for comorbidity. We updated the mapping of diagnosis codes to genes using OMIM as well as OrphaNet data [53] . The Mendelian diseases each have from one to 50 implicated genes ( Supplementary Fig. 1a ), except for the five chromosomally associated disorders, which we remove from further analysis. Of the complex diseases in the Blair analysis, 13 are cancers. We mapped 10 of these ICD code sets to 15 cancers included in TCGA ( Supplementary Data 2 ). Then, for all tumour types with both copy-number-alteration data and whole-exome sequencing data available, we download the calls of recurrently altered genes as assessed by the Broad Institute and made available in the Firehose ( http://www.broadinstitute.org/cancer/cga/Firehose ) download data set of 23 September 2013. MutSigCV assigns a statistic for evidence of selection for mutation of a gene across a set of tumours. For each tumour type, we select those genes with a q value statistic <0.25. GISTIC2 identifies genes in significantly recurrent and focal regions of copy-number amplification or deletion, and we include only the genes in copy-number peaks that contain fewer than 50 genes. Each tumour type has from zero to hundreds of associated genes either mutated or copy-number altered ( Supplementary Fig. 1b ). The other data used include the Entrez gene info data ( ftp://ftp.ncbi.nlm.nih.gov/gene/DATA/GENE_INFO/Mammalia/Homo_sapiens.gene_info.gz ), which was used to find common identifiers between all data sets, the BioGRID data ( BIOGRID-ORGANISM-Homo_sapiens-3.2.119.mitab.txt ), HumanNet data ( HumanNet.v1.join.txt ), the pathway gene set list from the Consensus Pathway Database and the FANTOM5 human gene expression data, which are described in the following section. Genetic similarity of comorbid diseases We test similarity of pairs of gene sets using a number of sources of evidence. Our similarity metrics are first evaluated on the aggregate of comorbid diseases to test the hypothesis that comorbidity is significantly related to shared genetic factors. Then, we use analagous tests for the pairs of diseases, to identify Mendelian disease and cancer with evidence of related gene sets. Below, we describe both uses of each metric. The gene enrichment metric scores the overlap of the Mendelian disease gene set of size m, within a cancer gene set of size c. The score assesses whether the number of genes in the overlap between the two sets is more than expected. For the per-pair score, we use a binomial model with success probability based on the fraction of all assayed genes that are in the Mendelian gene set , number of trials corresponding to the cancer recurrently mutated gene set size c, and number of successes corresponding to the size of the overlap between the sets. For the aggregate score, we test whether the number of genes shared across 427 pairs of Mendelian diseases and comorbid cancers is more than would be expected at random. Overall, 41 genes are shared in common between comorbid diseases. We assess whether 41 is a significantly elevated number by performing a simulated convolution of the 427 binomial tests: for each pair, the binomial model, as before, has a success probability based on the fraction of total genes that are Mendelian disease genes and a number of trials based on the number of recurrent cancer genes. Each model is simulated 100,000 times and the numbers for each pair are added to generate an expected distribution. We find that 41 occurs in 2.1% of random trials ( Supplementary Fig. 2a ) The pathway metric utilizes the NCI Pathway Interaction Database and the PharmGKB subsets of the Consensus Pathway Database to obtain a diverse and non-redundant set of pathways. The set contains 1,343 pathways and a total of 4,954 genes. We create a gene list containing the union of all genetically altered cancer genes across all of the cancers studied, and we remove all pathways with enrichment in this list to filter very general cancer cellular processes. We score strength of the overlap of a cancer gene set within each gene set associated with each remaining pathway using the same binomial gene-enrichment score, then corrected by the number of pathways with the Benjamini–Hochberg method [54] . Many pathways have no overlap with a cancer’s gene list, so the enrichment score for these is 1. For the Mendelian diseases, we consider a pathway to be affected if it contains any Mendelian disease gene. To assess the similarity for a pair of diseases, we use the Spearman correlation coefficient of the pathway scores for each disease across all pathways, with the Spearman significance statistic providing our per-pair score. For the aggregate score across comorbid pairs, we use a cutoff on cancer enrichment ( q value <0.1), and we count the number of pathways that are both enriched in the cancers and involved in the Mendelian disease. We find 136 pathways shared in comorbid pairs. We assess whether this number of overlapping pathways is more than expected using the convolution of hypergeometrics, similar to the gene-enrichment convolution (results shown in Supplementary Fig. 2b ). To ensure that the significance is not only owing to two Mendelian disorders with the most pathways impacted, we also run this test when Rubinstein–Taybi syndrome and Pervasive Specified Congenital Anomalies are removed: in this case only 81 pathways are shared but the overlap is still highly significant. The network metric measures the number of direct interactions of each Mendelian disease gene set with the cancer gene set. This number is compared with the number found in a set of shuffled networks, created using a degree-preserving randomization algorithm [55] . A pair of diseases is considered similar if fewer than 5% of random networks have the same or higher number of interactions. For the aggregate score, we count over the Mendelian diseases, the number of edges between a Mendelian disease's genes and the set of comorbid cancer genes. This count is compared against the count from the shuffled networks. We use two networks to independently score our disease pairs. In the BioGRID binary interaction data set, a curated set of genetic interations and protein interactions, there are 140,402 edges on 14,112 nodes, covering 86% of Mendelian disease genes and all but four of our Mendelian disease sets. In all, there are 797 direct edges between comorbid genes in this network, a number found in <2% of random networks. Another network, HumanNet, is constructed by integrating a number of data sources, and it assigns a confidence score to each learned interaction. We take the top 10% most confident edges, resulting in a network with 7,931 nodes and 47,934 edges. In HumanNet, there are 296 direct edges between comorbid disease genes, which is a number found in only 0.2% of random networks. To these pairwise and aggregate measures of similarity, we wished to add an entirely unbiased source of information on functional similarity and cell-specific expression. We developed a coexpression metric utilizing the data from FANTOM5. The FANTOM5 data covers a diverse range of 889 cellular states, assessing promoter activity in each gene in each cell or tissue type. We download the human CAGE peak data quantified by transcripts per million ( http://fantom.gsc.riken.jp/5/datafiles/latest/extra/CAGE_peaks/hg19.cage_peak_tpm_ann.osc.txt.gz ). Adding all the peaks that are assigned to the same gene, we create an estimate of aggregate expression of each gene in each sample. As we wish to measure whether genes involved in a pair of diseases are expressed in the same conditions, we calculate coexpression of pairs of genes using the Pearson correlation coefficient. To calculate our coexpression similarity for a pair of Mendelian disease and cancer, we consider that significantly elevated coxpression between any cancer gene and a set of Mendelian disease genes represents interesting similarity. Thus, for each cancer gene, we compare whether the set of Mendelian disease genes has high coexpression with that cancer gene, as compared against the distribution of coexpression of all other genes with the cancer gene. We test this for each cancer gene using the Wilcoxon rank-sum test. The P values are then corrected for the number of cancer genes tested using the Benjamini–Hochberg method. For each metric, we correct the pairwise similarity scores by the number of comorbid pairs examined, to create our list of interesting disease pairs. The scores are shown in Supplementary Data 3 and 4 . We find that comorbid Mendelian disease and cancer are more likely to have genetic similarity by the pairwise metrics. To assess the influence of the number of annotated Mendelian genes on detection of genetic similarity and comorbidity, we performed L1 regularized logistic regression using models with and without the number of Mendelian genes as an explicit covariate. Logistic regressions were performed in python using the scikit-learn package. The results are shown in Supplementary Fig. 6 . Cancer gene-expression analysis For melanoma and lower-grade gliomas, level 3 RNASeq data were downloaded from the TCGA portal, and the RSEM [56] expected counts were rounded to create the input to the analysis. For the albinism analysis, we aggregate all melanoma patient data into a count matrix, which we then transform using the variance stabilizing transformation from DESeq2 (ref. 57 ), which is recommended for clustering data. Then, we apply consensus clustering using the ConsensusClusterPlus [58] package, and an optimum clustering is found (based on change in classification consistency) of k =4. Three main large clusters are consistent through k =3 to k =6. We use the R package Survival [59] to assess survival difference between the groups and to plot, based on the available TCGA clinical data. For the ectodermal dysplasia analysis, we use TCGA barcodes (01 for primary tumour, and 06 or 07 for metastasis), to identify the metastasis and primary samples. We use edgeR to calculate library size factors and estimate dispersion, followed by assessment of differential expression. For the gene set analysis, we use voom [60] to transform the data, allowing use of the camera gene set score [61] . In addition, we use the limma [62] differential expression t-statistic to form a pre-ranked input to GSEA [63] for gene set differential expression analysis. In the lower-grade glioma analysis, we use the copy-number and exome-sequencing data that match the expression data to identify cases with VENTX deletion and cases with IDH1 mutation. We aggregate the expression data for all patients with available matched mutation and copy-number data, and we use the limma voom function to transform the expression data. We create a gene set containing the candidate holoprosencephaly genes, and then, as above, we use voom, camera and GSEA to analyse the gene set differential expression. Availability of code for reproducibility All source data used, code to create the tables, and output tables can be accessed at http://bit.ly/melamed_comorbidity , allowing full reproducibility of results. How to cite this article: Melamed, R.D. et al. Genetic similarity between cancers and comorbid Mendelian diseases identifies candidate driver genes. Nat. Commun. 6:7033 doi: 10.1038/ncomms8033 (2015).